Reliable detection of subclonal single-nucleotide variants in tumour cell populations According to the clonal evolution model, tumour growth is driven by competing subclones in somatically evolving cancer cell populations, which gives rise to genetically heterogeneous tumours. Here we present a comparative targeted deep-sequencing approach combined with a customised statistical algorithm, called deepSNV, for detecting and quantifying subclonal single-nucleotide variants in mixed populations. We show in a rigorous experimental assessment that our approach is capable of detecting variants with frequencies as low as 1/10,000 alleles. In selected genomic loci of the TP53 and VHL genes isolated from matched tumour and normal samples of four renal cell carcinoma patients, we detect 24 variants at allele frequencies ranging from 0.0002 to 0.34. Moreover, we demonstrate how the allele frequencies of known single-nucleotide polymorphisms can be exploited to detect loss of heterozygosity. Our findings demonstrate that genomic diversity is common in renal cell carcinomas and provide quantitative evidence for the clonal evolution model. Cancer is a somatic evolutionary process in which mutations render cells non-cooperative and overly proliferative [1] , [2] , [3] . Selectively advantageous driver mutations accumulate in multiple rounds of clonal expansions together with hitch-hiking, selectively neutral passenger mutations [1] , [4] . The driving forces of evolution include mutations in single cells and selection of the most proliferative clones. Mutation diversifies an evolving population by generating novel variants, whereas selection has a purifying effect. Genomic diversity resulting from the interplay of mutation and selection is thus a key signature of evolution. Studying genomic diversity in heterogeneous cell populations became possible with second-generation sequencing technologies that process millions of DNA molecules in a single run [5] . They enable direct sequencing of mixed samples, such as virus populations [6] , [7] , bacterial communities [8] , tumours [9] , [10] , [11] and pooled samples [12] , [13] , and the reconstruction of their genomic composition. However, single-nucleotide errors resulting from target enrichment, library preparation and base calling are frequent on all current sequencing platforms [5] , and they are difficult to separate from true low-frequency single-nucleotide variants (SNVs). Sequencing error rates vary across genomic sites, often reaching up to 1%, and they challenge accurate calling of SNVs present at frequencies below this rate. To overcome these limitations, we employ a comparative sequencing strategy, where the same genomic region is compared between a heterogeneous test sample and a homogeneous control sample, using a customised statistical algorithm ( Fig. 1a ). The control sample allows for estimating the local error rate, which increases the power for calling true variants at a given false-positive rate. Unlike true variants, sequencing errors depend on the directionality of sequencing and tend to occur more often on one DNA strand than the other, which can be used to further increase the specificity of variant calling [14] , [15] . Batch-library preparation and sequencing in the same run ensure identical noise characteristics of test and control, an important prerequisite for reliable variant detection. 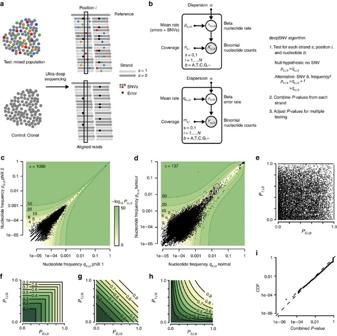Figure 1: Testing for low-frequency SNVs with deepSNV. (a) For a mixed sample, the distribution of reads with SNVs (grey arrows with coloured dots) resembles the population structure, but sequencing errors (black dots) confound calling of SNVs. A homogeneous control sample allows for precise estimation of the local error rate, which is often biased to one strand, and enables accurate SNV calling against the background noise frequency. (b) Generative probabilistic model underlying deepSNV and summary of the algorithm. At each positioniin the test experiment and for each strands, the frequency of nucleotideb, πs,i,b, is drawn from a beta distribution with meanps,i,b. The dispersion α quantifies the variability of the nucleotide frequencies across experiments. In the absence of an SNV,ps,i,bresembles the error rates. The nucleotide countsXs,i,bare modelled by a binomial distribution with coveragens,i. The same model is used for generating the nucleotide countsYs,i,b. in the control experiment with mean error rateqs,i,b. Testing for an SNVbat positioniamounts to test the null hypothesis that the mean relative frequencies of nucleotidebare identical in test and control experimentps,i,b=qs,i,b. (c) Scatter plot of mean nucleotide frequencies from strand 0 for two phiX replicates (black dots). Colours and contour lines denote the strand-specificP-value of deepSNV for median coverage of 166,000. (d) Scatter plot of nucleotide frequencies for a cancer sample and control (black dots). Contour lines are shown for the median control coverage of 42,438. (e) Scatter plot ofP-values from both strands of the two phiX replicates. (f–h) CombiningP-values. Contours of the jointP-value for the max (f), average (g) and product (h) statistic. (i) Empirical distribution of jointP-values for the two phiX experiments, combined with the max method. Figure 1: Testing for low-frequency SNVs with deepSNV. ( a ) For a mixed sample, the distribution of reads with SNVs (grey arrows with coloured dots) resembles the population structure, but sequencing errors (black dots) confound calling of SNVs. A homogeneous control sample allows for precise estimation of the local error rate, which is often biased to one strand, and enables accurate SNV calling against the background noise frequency. ( b ) Generative probabilistic model underlying deepSNV and summary of the algorithm. At each position i in the test experiment and for each strand s , the frequency of nucleotide b , π s,i,b , is drawn from a beta distribution with mean p s,i,b . The dispersion α quantifies the variability of the nucleotide frequencies across experiments. In the absence of an SNV, p s,i,b resembles the error rates. The nucleotide counts X s,i,b are modelled by a binomial distribution with coverage n s,i . The same model is used for generating the nucleotide counts Y s,i,b . in the control experiment with mean error rate q s,i,b . Testing for an SNV b at position i amounts to test the null hypothesis that the mean relative frequencies of nucleotide b are identical in test and control experiment p s,i,b = q s,i,b . ( c ) Scatter plot of mean nucleotide frequencies from strand 0 for two phiX replicates (black dots). Colours and contour lines denote the strand-specific P -value of deepSNV for median coverage of 166,000. ( d ) Scatter plot of nucleotide frequencies for a cancer sample and control (black dots). Contour lines are shown for the median control coverage of 42,438. ( e ) Scatter plot of P -values from both strands of the two phiX replicates. ( f – h ) Combining P -values. Contours of the joint P -value for the max ( f ), average ( g ) and product ( h ) statistic. ( i ) Empirical distribution of joint P -values for the two phiX experiments, combined with the max method. Full size image deepSNV algorithm Comparing test and control experiment requires estimation of inter-experimental variation. For each genomic position, we model the number of observed nucleotide counts on the two strands in both experiments with a hierarchical binomial model and derive a likelihood ratio test for each base to quantify the excess of the SNV in the test over the control sample ( Fig. 1b–d; Methods). We aggregate the test results from both strands into a single P -value that quantifies how likely it is that an observed nucleotide is a sequencing error, rather than a true variant ( Fig. 1e–i ). P -values are corrected for the number of tests performed, controlling either the family-wise error rate (FWER; Bonferroni method) or the false discovery rate (FDR; Benjamini–Hochberg) [16] . We have implemented the testing procedure in the R package 'deepSNV', which is freely available at http://www.bioconductor.org . Experimental analysis of specificity and sensitivity An initial analysis of two Illumina GAII x sequenced replicates of the phiX genome confirmed the accuracy of the P -values computed by deepSNV as a measure of type-1 errors ( Fig. 1i ). Accurate P -values are critical, because the algorithm assesses all four minor alleles on each position in the genome, resulting in thousands or even millions of tests, and multiple testing schemes fail if P -values are biased. Specificity is lost if sequencing is performed in different runs because of dissimilar error distributions, but can partially be recovered by data normalisation ( Supplementary Fig. S1 ). To assess the power of comparative sequencing followed by variant calling by deepSNV, we generated synthetic test samples by mixing six plasmids containing known clones of a 1.5 kb fragment of the HIV pol gene at relative frequencies 10 −5 , 10 −4 , 10 −3 , 10 −2 and 10 −1 , respectively, together with a majority clone at frequency 0.89999 ( Supplementary Table S1 ). The majority clone also served as a control sample. The five low-frequency clones contained approximately 100 SNVs relative to the control clone. As some variants are present on multiple clones and can be masked by clones with higher frequencies, the number of unique variants is between 36 and 101 ( Table 1 ). PCR target enrichment was simulated by amplifying the inserts from the two samples and resulted in elevated noise levels, but only minimally altered variant frequencies ( Supplementary Fig. S2 ). Both PCR-amplified and non-amplified mixture and control samples were sequenced at 69,203 to 117,180× coverage on an Illumina GAII x sequencer in the same lane using barcodes and 36 nucleotide reads ( Supplementary Table S2 ). Reads were aligned to the HXB2 HIV reference genome to avoid bias towards any of the clones. At each position, nucleotides with Phred quality larger than 25 were counted, insertions and alignment artifacts were ignored, and 23 variants of a confirmed subpopulation in the control sample were masked ( Supplementary Fig. S3 ). Table 1 Comparison of SNV calling methods. Full size table For SNV frequencies larger than or equal to 10 −4 , the measured nucleotide frequencies accurately agree with the true values, whereas SNVs with frequencies below 10 −4 are additively biased by sequencing errors that occurred at a median rate of 2.2×10 −5 ( Fig. 2a ). The long tail of sequencing errors confounds SNV calling, but this limitation can partially be overcome by testing against the control ( Fig. 2b ). 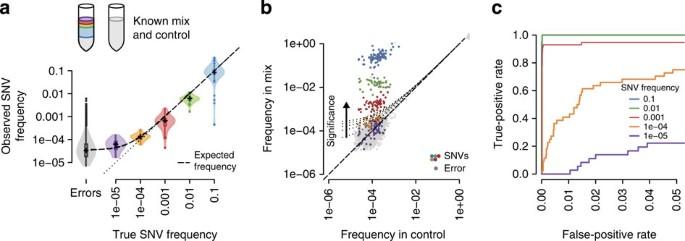Figure 2: Experimental assessment of deepSNV. (a) Observed frequency distributions for SNVs and sequencing errors in a test data set of known composition. The dashed line shows the expected frequency based on an additive error model. (b) Scatter plot of nucleotide frequencies in control and mixture sample, and indicated levels of significance of the deepSNV test. The null hypothesis of the test implies that the observed relative frequencies lie close to the diagonal, whereas the alternative allows the frequency in the test experiment to be greater than in the control. (c) Receiver-operating characteristic curves demonstrate high power at low false-positive rates. Figure 2: Experimental assessment of deepSNV. ( a ) Observed frequency distributions for SNVs and sequencing errors in a test data set of known composition. The dashed line shows the expected frequency based on an additive error model. ( b ) Scatter plot of nucleotide frequencies in control and mixture sample, and indicated levels of significance of the deepSNV test. The null hypothesis of the test implies that the observed relative frequencies lie close to the diagonal, whereas the alternative allows the frequency in the test experiment to be greater than in the control. ( c ) Receiver-operating characteristic curves demonstrate high power at low false-positive rates. Full size image DeepSNV calls variants with frequencies higher than 10 −4 with high sensitivity and specificity ( Fig. 2c ). At an FDR of 0.05, it recovered all SNVs of frequency 10 −1 and 10 −2 , 53/57 variants of frequency 10 −3 , and 3/44 variants of frequency 10 −4 , whereas the false-positive rate was 2/5,740 ( Table 1 ). With a more conservative FWER control, no false positives were called. At a fixed FWER, deepSNV outperformed all related software packages [17] , [18] , [19] in terms of both specificity and sensitivity. Although the power of deepSNV is comparable to that of vipR for variant frequencies of 0.1 and 0.01, its performance is considerably better for variant frequencies of 0.001 and 0.0001 ( Supplementary Fig. S4 ). Most importantly, deepSNV achieves a high sensitivity for small false-positive rates, but also a high overall power as measured by the area under the receiver-operating characteristic (ROC) curve ( Supplementary Table S3 ). With the exception of VarScan [17] , however, deepSNV is the only method specifically designed for detecting SNVs in mixed populations with an unknown number of clones. For low frequencies of 10 −3 , deepSNV achieves a power of 86%, compared with the second-best method with 53%. Our algorithm was also the fastest because of a direct C interface to the condensed bam alignments that present a bottleneck for nucleotide-wise analysis. The deepSNV algorithm uses a Phred quality cutoff to avoid false positives caused by ambiguous nucleotide calls. The choice of the cutoff has a negligible effect on performance as long as it is greater than 10 ( Supplementary Fig. S5A ). For higher cutoffs, there is a small decrease in power because of the reduced coverage. A default Phred score cutoff of 25 resulted in a good compromise between specificity and sensitivity. The performance of deepSNV was also found not to depend strongly neither on the chosen method of P -value combination, nor on PCR amplification ( Supplementary Table S4 ). Power calculations show that additional sensitivity for calling low-frequency variants can be gained by increased sequencing depth ( Supplementary Fig. S5B ). Roughly, the required coverage for calling a variant needs to be at least ten times higher than its inverse frequency. For large genomes, the power of SNV calling is diminished by multiple testing corrections, but it remains high for variants present in 1/1,000 alleles ( Supplementary Fig. S5C ). Subclonal diversity in renal cell carcinomas We extracted 10,374 bp of the VHL , PTEN , TP53 and CDKN1B genes by PCR from matched normal and tumour samples of four clear cell renal cell carcinoma (RCC) patients and sequenced the fragmented amplica at ultra-deep coverage ( Fig. 3a and Supplementary Tables S5–S7 ). For one patient, additional samples from an opposing side of the primary tumour and from a metastatic lesion were taken, and an additional 4,378 bp of the PTEN gene were isolated by PCR. We detected a total of 24 (range 1–13 per sample) different SNVs in the tumours with frequencies ranging from 0.0002 to 0.34, as opposed to only two variants with higher frequencies in the controls (FWER < 0.05, beta-binomial test; Table 2 and Fig. 3b ). Eight selected subclonal variants were resequenced and confirmed on a Roche GS Junior sequencer using 300 bp reads ( Supplementary Table S8 ). The validation experiment also showed an accurate agreement of the nucleotide frequencies with the original discovery experiment ( Fig. 3c ). The nucleotide substitution spectrum is similar to previous reports in RCC [20] ( Fig. 3d ), with a characteristic overrepresentation of {C,G}>{T,A} deaminations at CpG dinucleotides and more prevalent G>A substitutions on the transcribed strand. 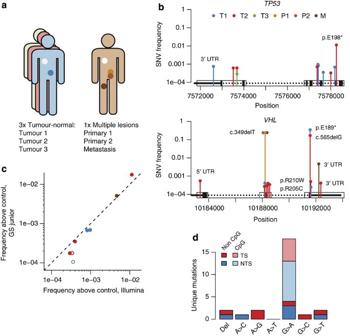Figure 3: Detecting intra-tumour heterogeneity in renal cell carcinomas. (a) Three matched tumour-normal samples and one case with biopsies from multiple lesions were analysed. (b) Distribution of SNV frequencies on theTP53(top) andVHL(bottom) genes. The colour represents the tumour sample. Black boxes indicate the PCR amplicons used, grey bars are exons. Only non-synonymous exonic SNVs are annotated. UTR, untranslated region. (c) A total of 8 of 23 subclonal SNVs detected by Illumina sequencing were validated by additional sequencing on a Roche GS Junior sequencer. Shown are the differences in the nucleotide frequencies, averaged from both strands, between the tumour and the control samples in the two experiments. Filled circles denote statistical significance (P<0.05; deepSNV test). (d) Distribution of base substitutions. NTS, non-transcribed strand, TS, transcribed strand. Figure 3: Detecting intra-tumour heterogeneity in renal cell carcinomas. ( a ) Three matched tumour-normal samples and one case with biopsies from multiple lesions were analysed. ( b ) Distribution of SNV frequencies on the TP53 (top) and VHL (bottom) genes. The colour represents the tumour sample. Black boxes indicate the PCR amplicons used, grey bars are exons. Only non-synonymous exonic SNVs are annotated. UTR, untranslated region. ( c ) A total of 8 of 23 subclonal SNVs detected by Illumina sequencing were validated by additional sequencing on a Roche GS Junior sequencer. Shown are the differences in the nucleotide frequencies, averaged from both strands, between the tumour and the control samples in the two experiments. Filled circles denote statistical significance ( P <0.05; deepSNV test). ( d ) Distribution of base substitutions. NTS, non-transcribed strand, TS, transcribed strand. Full size image Table 2 SNVs in tumor samples. Full size table In three out of four cases, the VHL gene was hit by a high-frequency truncating mutation, namely a stop codon at p.E189* at frequency 0.34 in tumour 1, and two single-nucleotide deletions, c.565delG and c.349delT, observed at frequencies 0.17 and 0.24 in tumour 2 and in the multiple lesions samples, respectively. The remaining 21 subclonal variants had low frequencies. Four subclonal SNVs were found in coding regions, of which one SNV at frequency 0.01 in tumour 2 introduces a stop codon in TP53 at p.E198. Another four SNVs occur in 3′- and 5′- untranslated regions. The remaining 13 variants are located in intronic regions. The co-occurrence of two intronic SNVs at 20-bp distance in tumour 1 (chr17: 7577407A>C and chr17: 7577427G>A) was detected both in the discovery experiment using Illumina and in the validation experiment using 454/Roche. All other SNVs sequenced on the same amplica were detected on separate alleles. The number of SNVs was much greater in tumour 1 ( n =13) and tumour 2 ( n =8) than in the other samples that contained only one or two SNVs. The estimated nucleotide frequencies may be utilised to infer regions of lost heterozygosity. For this purpose, the frequencies of germline single-nucleotide polymorphisms (SNPs) were assessed. The difference of the SNP allele frequencies in the normal versus tumour samples measures the excess of an allele that indicates lost heterozygosity ( Fig. 4a–c ). With this approach, we detected loss of parts of chromosome 3 in five out of six samples, including the multiple-lesions cases. The copy-number losses were confirmed by standard copy-number analysis using 250-kb SNP arrays in three matched tumour-normal samples ( Fig. 4d–f ). 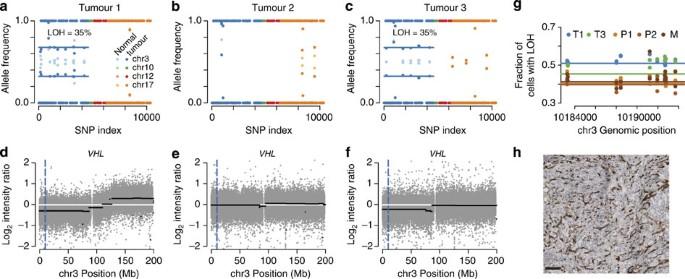Figure 4: Detecting copy-number alterations from SNP imbalances. (a–c) Allele frequencies of known SNPs in matched tumour-normal samples. (a) Tumour 1, (b) tumour 2, (c) tumour 3. Light colours denote the frequency in the normal control, dark colours denote the frequency in the tumour. A deviation from heterozygous SNP frequencies of 0.5 indicates loss of heterozygosity (LOH). (d–f) Copy number profiles and logarithmic probe intensities of 1 M SNP arrays for the samples presented in panel (a–c). (g) Fraction of cells with LOH. The difference of heterozygous SNP frequencies on chromosome 3 (chr3) allows for computing the number of cells carrying only one copy. The resulting fraction of 43% is conserved across the three tumour samples of the same patient. (h) Histology of RCC. CD34-positive, non-cancerous cells (brown) in the primary RCC tissue sample. Nuclei are stained blue. The scale bar denotes 100 μm. Figure 4: Detecting copy-number alterations from SNP imbalances. ( a – c ) Allele frequencies of known SNPs in matched tumour-normal samples. ( a ) Tumour 1, ( b ) tumour 2, ( c ) tumour 3. Light colours denote the frequency in the normal control, dark colours denote the frequency in the tumour. A deviation from heterozygous SNP frequencies of 0.5 indicates loss of heterozygosity (LOH). ( d – f ) Copy number profiles and logarithmic probe intensities of 1 M SNP arrays for the samples presented in panel ( a–c ). ( g ) Fraction of cells with LOH. The difference of heterozygous SNP frequencies on chromosome 3 (chr3) allows for computing the number of cells carrying only one copy. The resulting fraction of 43% is conserved across the three tumour samples of the same patient. ( h ) Histology of RCC. CD34-positive, non-cancerous cells (brown) in the primary RCC tissue sample. Nuclei are stained blue. The scale bar denotes 100 μm. Full size image The SNP allele counts also allow for estimating the fraction of cells with a lost allele, which can indicate a mixture of normal and tumour cells ( Fig. 4g ). We estimated a tumour content of 42 to 50%. In the case of multiple lesions per patient, the tumour content was conserved across the three samples, which suggests a constant, stable equilibrium between tumour and normal cells ( Fig. 4h ). The frequency of hemizygous SNPs in all three cases with loss-of-heterozygosity (LOH) agrees well with the mutation frequencies of truncating VHL mutations, suggesting that both alleles of this tumour suppressor gene are impaired in tumour cells. Taken together, the clonal VHL point mutation and loss of chromosome arm 3p as well as the 7 subclonal mutations found at the time of diagnosis suggest, for tumour 1, the evolutionary history summarised in Fig. 5 . 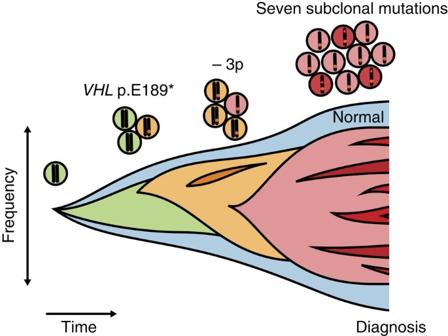Figure 5: Possible evolutionary history of tumour 1. A point mutation inVHLoccurred at early stages with a subsequent loss of chromosome arm 3p, each followed by a selective sweep. At the time of diagnosis, seven subclonal mutations are observable in theVHLandTP53genes. Figure 5: Possible evolutionary history of tumour 1. A point mutation in VHL occurred at early stages with a subsequent loss of chromosome arm 3p, each followed by a selective sweep. At the time of diagnosis, seven subclonal mutations are observable in the VHL and TP53 genes. Full size image We have presented a comparative targeted deep-sequencing approach and a powerful statistical algorithm for detecting subclonal SNVs in heterogeneous cell populations. The specificity and sensitivity of the method have been rigorously assessed on multiple control experiments. Its reliability results from an overdispersed statistical model of nucleotide counts and from integrating the signals from both DNA strands. The current limit of detection is around 1/10,000 alleles, but it may be further improved by increased coverage and higher sequencing fidelity with improved biochemistry or barcoded reads [21] . The method can be applied to any tissue sample of a heterogeneous cell population for which a control sample is available. It may be utilised for the analysis of pathogen populations, such as viruses or bacteria, for the assessment of T-cell diversity [22] , or for detecting rare somatic mutations associated with diseases, such as the Proteus syndrome [23] . Another application is the cost-effective pooled sequencing of multiple individuals. In cases where a pure sample of the majority clone is not available, a closely related reference sample could be used as a control, for example, a stock plasmid of the genomic regions of interest. The deepSNV algorithm has primarily been designed for targeted sequencing of selected loci at ultra-deep coverage, but power calculations indicate that the algorithm can also detect heterozygous mutations at 100× coverage in comparative exome-sequencing studies, and simulations show that this application is computationally feasible. We have demonstrated the utility of the sequencing approach for RCC tissue samples, revealing multiple subclonal variants and intra-tumour heterogeneity on the chromosomal and single-nucleotide level. In addition, the imbalances of SNP allele frequencies were used to correctly predict an LOH on chromosome 3 in only a subset of the tumour samples. Recent studies found genomic heterogeneity in breast cancer [10] , [24] , pancreatic cancer [25] , [26] , and B-cell chronic lymphocytic leukemia [9] , as well as mosaic amplifications of tyrosine kinase receptor genes in glioblastoma [27] . Together, these findings provide compelling evidence for clonal evolution as a general mechanism in cancer development. Quantifying subclonal diversity in tumours is important for understanding the driving forces of their evolution, and sensitive methods are required for detecting low-frequency drug-resistant mutations before treatment [28] . Most tumour variants were found at frequencies below 1/1,000 alleles. This observation agrees with the notion that mutations occur initially in single cells and selection amplifies few alterations to high frequencies, which causes the number of different variants to decrease with increasing frequencies. A total of 13 out of 21 subclonal variants occurred in introns, and they are most likely neutral-passenger mutations. All SNVs were found in the VHL and TP53 genes, which show a similar dinucleotide composition as the PTEN and CDKN1B amplicons, and made up 8,753 of the 10,375 bp sequenced in each sample, suggesting an overrepresentation of subclonal SNVs in VHL and TP53 ( P =0.06, Fisher's exact test) that requires further investigation. As the majority of variants is intronic and appears to be selectively neutral, a possible explanation might be an increased mutation rate at these loci, but additional experiments comprising more genes in a larger cohort are necessary to test this hypothesis. An overall elevated mutation rate may also explain that two RCC cases showed a substantially larger number of low-frequency SNVs than the other samples. An extrapolation of our findings from the selected loci to the entire genome suggests that there are more than 100,000 subclonal SNVs present in a tumour cell population of comparable size. This substantial intra-tumour genomic diversity could have important consequences for cancer diagnosis and it may directly impact treatment strategies [29] . deepSNV algorithm The nucleotide counts in the test experiment X s,i,b, b {A,T,C,G,−}, at genomic position i on strand s =0,1 (forward, reverse), are modelled by a hierarchical binomial model with coverage n s,i and substitution rates drawn from a beta distribution with mean p s,i,b and parameter α : Here, the gap symbol ('−') is treated as a fifth nucleotide character (see Fig. 1b for a graphical depiction). The marginal counts of nucleotide b follow a beta-binomial distribution, Here, the beta-binomial distribution is parameterised by the mean p s,i,b , and dispersion α. For small p s,i,b , the variance of the nucleotide count is . The overdispersion adds a quadratic term to the variance, which vanishes for large values of α (compare Fig. 1c and d ). In this limit, one recovers a binomial model with variance proportional to the mean. Similarly, we define Y s,i,b as the count of nucleotide b at position i and strand s in the control experiment with coverage m s,i , In the absence of an SNV, the substitution rates of non-consensus bases are identical, p s,i,b = q s,i,b , and reflect sequencing errors only, whereas in the presence of an SNV b with frequency f in the test experiment, the rate p s,i,b = q s,i,b + f is greater than the error rate q s,i,b . The deepSNV algorithm detects SNVs by testing the alternative hypothesis H 1 : p s,i,b > q s,i,b against the null-hypothesis H 0 : p s,i,b = q s,i,b for each locus, nucleotide, and strand by means of a likelihood ratio test statistic Here, g denotes the probability mass function of the beta-binomial distribution, are the method-of-moments estimates of the mean nucleotide rates under H 1 , and the estimated mean rate under H 0 . The estimate of the dispersion is computed by numerical maximisation of the log-likelihood under H 0 , . Under the null-hypothesis and for large coverages, D s,i,b is χ 2 1 -distributed with one degree of freedom, as the models are nested, H 0 H 1 . A P -value is computed as P s,i,b =1− G ( D s,i,b ), where G is the cumulative distribution function of the χ 2 2 distribution. The resulting two P -values for each strand P 0,i,b and P 1,i,b can be combined in different ways into a single P -value, depending on which violation of the joint null-hypothesis is characteristic of true SNVs. The joint P -value P i,b denotes the probability that the observed combination of nucleotide counts on both strands resulted from sequencing errors. It is defined as the tail probability of a given combination of P -values Q i,b ( P 0,i,b , P 1,i,b ) under the null-hypothesis that the P -values of both strands are independently uniformly distributed. The maximum statistic Q i,b= max{ P 0,i,b , P 1,i,b } generates a joint P -value of P i,b= max{ P 0,i,b , P 1,i,b } 2 as a joint P -value ( Fig. 1f ). The average statistic Q i,b= ( P 0,i,b + P 1,i,b )/2 yields P i,b =( P 0,i,b + P 1,i,b ) 2 if P 0,i,b + P 1,i,b <1 and (1− P 0,i,b − P 1,i,b ) 2 else ( Fig. 1g ). A third alternative is Fisher's method [30] , which is based on the product of the two P -values Q i,b = P 0,i,b × P 1,i,b , the negative logarithm of which then follows χ 2 2 -distribution ( Fig. 1h ). The algorithm tests in total N ×4 genomic sites, where N denotes the length of the sequence and 4 equals the size of the alphabet minus 1, as the consensus base is excluded from the test. The combined P -values are thus corrected for multiple testing by either the method of Bonferroni or Benjamini–Hochberg [31] for a control of the FWER or the FDR, respectively. To avoid false positives arising from bad nucleotides, the algorithm can be adjusted to only consider calls above a Phred threshold, which was set to 25. Detection of LOH and tumour content from SNP frequencies LOH skews the allele-frequency ratios of heterozygous SNPs in tumour samples, which are typically a mixture of tumour and normal cells. Suppose there exists a heterozygous SNP with alleles A and a in the sample. Ideally, the ratio of A and a alleles would be r=f A / f a =1. If the tumour population has lost allele a , then the frequency of A to a alleles changes to r= (1−ρ)−1, where ρ is the fraction of tumour cells. In the case of aneuploidy of degree n in allele a , the fraction of cells with LOH, that is, tumour cells, can be estimated as ρ= [ r −1]/[ r +( n −1)]. In the presence of sequencing bias, the observed ratio of allele A over a is altered. If, for a heterozygous SNP, the true ratio is known to be one, then the bias can be estimated from a control experiment as the inverse allele ratio 1/ r 0 . Thus, the corrected tumour fraction is ρ= [ r/r 0 −1]/[ r/r 0 +( n −1)]. For a simple LOH ( n= 1), the corrected tumour fraction is ρ= 1− r 0 / r . Experimental test data Six 1.5 kb variants of the HIV pol gene were cloned, sequenced with Sanger sequencing, and mixed at frequencies 10 −5 , 10 −4 , 10 −3 , 10 −2 , 10 −1 and 0.89999, respectively. A pure sample of the majority clone served as the control. Both samples were additionally amplified by 25 cycles of PCR. The resulting four samples were fragmented, adaptor-ligated and sequenced with barcodes in a single lane of an Illumina GAIIx sequencer. The resulting reads were aligned to the HXB2 reference with novoalign version 2.07.10 ( www.novocraft.com ). Comparison of methods The performance of deepSNV on the test data was compared with VarScan 2.2.5 (ref. 17 ), CRISP, [18] v5 and vipR [19] 0.0.11. For each algorithm, the minimal base quality was set to 25, and only variants from both strands were accepted. The minimal variant frequency was set to 1/10,000 (VarScan) and the poolsize was set to 10,000 (CRISP, vipR). ROC curves and the area under the ROC curve were computed for each variant frequency with the R package ROCR [32] . See Supplementary Methods for a detailed description of the chosen options. Power calculations The power of the deepSNV algorithm was assessed as a function of sequencing depth, genome size and minimal Phred nucleotide quality. For coverage smaller than the observed, the power of deepSNV was computed by sub-sampling without replacement from the actual nucleotide counts. For higher coverage, error rates π s,i,b were drawn independently for each genomic locus from a Dirichlet distribution trained across all observed sites. The nucleotide counts X s,i,b and Y s,i,b were sampled from multinomial distributions with mean coverage of the test and control experiments, respectively. To quantify the loss of power introduced by Benjamini–Hochberg multiple-testing correction, we sampled the distribution of P -values 20 times, corrected each sample for a given number of tests, and averaged the results. For the Bonferroni method, no sampling was performed; instead the P -values were directly adjusted to the number of tests imposed by a given genome size. The effect of the Phred quality cutoff was measured by varying the threshold at increments of 5 from 0 to 35 on the actual data and computing the power for each threshold. RCC samples This study was approved by the local commission of ethics (reference number StV 38-2005). Four fresh-frozen samples, including normal tissue, from a single metastatic RCC patient and matched tumour-normal samples from three other RCC patients were analysed. Approximately 50 μg of genomic DNA was isolated from each sample and selected loci were amplified with 33 cycles of PCR using a total of at least 100 ng genomic DNA as template. The amplica were pooled according to their length, fragmented, adaptor-ligated and sequenced on separate lanes of an Illumina GAII x sequencer (multiple lesions case) with 76 bp single-end reads or on a single lane of an HiSeq2000 sequencer with barcoded adaptors and 36 bp single-end reads. Reads were aligned to the UCSC hg18 human reference (multiple lesions) or the UCSC hg19 reference with novoalign 2.07.10 ( Supplementary Methods ). Subclonal variant validation Eight subclonal SNVs were selected for validation on a Roche GS Junior sequencer. A total of four PCR amplicons approximately 300 bp long were extracted from 100 ng template DNA with primers containing sequencing adaptors. For TP53 exon 7 and VHL exon 2, the corresponding amplicon used for Illumina sequencing served as PCR template, whereas in the other two cases primary tumour DNA was used. Reads were aligned using Mosaik ( http://bioinformatics.bc.edu/marthlab/Mosaik ) to the hg19 human genome. Accession codes: The sequencing data have been deposited in the European Nucleotide Archive under accession number ERP001312 . How to cite this article: Gerstung, M. et al . Reliable detection of subclonal single-nucleotide variants in tumour cell populations. Nat. Commun. 3:811 doi: 10.1038/ncomms1814 (2012).